In vivoassessment of human brain oscillations during application of transcranial electric currents Brain oscillations reflect pattern formation of cell assemblies’ activity, which is often disturbed in neurological and psychiatric diseases like depression, schizophrenia and stroke. In the neurobiological analysis and treatment of these conditions, transcranial electric currents applied to the brain proved beneficial. However, the direct effects of these currents on brain oscillations have remained an enigma because of the inability to record them simultaneously. Here we report a novel strategy that resolves this problem. We describe accurate reconstructed localization of dipolar sources and changes of brain oscillatory activity associated with motor actions in primary cortical brain regions undergoing transcranial electric stimulation. This new method allows for the first time direct measurement of the effects of non-invasive electrical brain stimulation on brain oscillatory activity and behavior. Understanding of the role of brain oscillations in human cognition and behavior has substantially advanced in the last decade [1] , [2] . Specific features of brain oscillations, such as amplitude [3] and phase [4] , are causally linked to brain functions and showed to be fundamental for perception, cognition and learning [2] , often disturbed in neurological or psychiatric diseases [5] . In this context, brain oscillatory activity was shown to be closely related to specific neurochemical processes [6] and short-range and long-range cortico-cortical communication [7] , [8] . Thus, brain oscillations represent a potential target for controlled interventions aiming at modulation of brain function [9] (neuromodulation). Such interventions include the application of extracranial electric currents to the human brain in order to modify brain function. However, in vivo effects of electrical brain stimulation on oscillatory activity are unknown, as electromagnetic noise generated by electrical stimulation blocks accurate recording of neurophysiological signals. Knowledge of the effects of electrical stimulation on brain oscillations would yield a better understanding of brain functions and may lead to improvements in treatment protocols related to brain stimulation for patient populations with neurological and psychiatric diseases [10] , [11] . A well-tolerated form of electrical brain stimulation is transcranial direct current stimulation (tDCS), which was shown to modulate brain activity at weak stimulus intensities (0.1–2 mA) [12] , [13] . tDCS has polarity-dependent effects on brain excitability [13] , and can influence cognition [14] , motor function [15] , learning [16] and memory consolidation [17] , [18] . Over the last two decades, tDCS has become increasingly used in the treatment of neurological and psychiatric diseases [19] , such as stroke [20] , depression [21] and dementia [22] . The influence of tDCS on millisecond-by-millisecond brain oscillatory activity is not known. Work using positron emission tomography (PET) and functional MRI (fMRI) [23] , [24] is incapable of providing the temporal resolution needed to test the hypotheses evaluated in this investigation [25] , [26] , [27] . Similarly, electroencephalography (EEG) has a limited capability of localizing underlying source generators due to its dependency on volume conduction boundaries, including the poorly conducting skull. Additionally, any conductive agents used with the EEG electrodes may not contact the stimulating electrodes as this would lead to saturation of the EEG amplifiers with the risk of damaging the EEG system. Thus, we used magnetoencephalography (MEG) as a tool to evaluate oscillatory activity, as it provides high-temporal resolution and also overcomes the limitations of EEG. MEG is a non-invasive technique that measures neuromagnetic activity in the range of femtoTesla (fT) and is nearly independent of the distorting effects of biological conduction boundaries like the scalp [28] . MEG sensors are superconducting quantum interference devices (SQUIDs) [29] organized in a helmet-shaped high-density array that covers the human head ( Fig. 1a ). 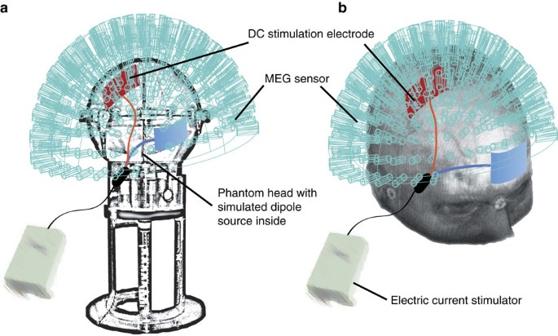Figure 1: Schematic illustration of the experimental setup. Magnetoencephalographic (MEG) recordings were performed with a phantom head (a) and healthy human volunteers (b). The electric stimulator was located outside the shielded MEG room and delivered 1 mA. The distance between the electric stimulation electrodes and the MEG sensor array (turquoise tubes) was 2–6 cm. Figure 1: Schematic illustration of the experimental setup. Magnetoencephalographic (MEG) recordings were performed with a phantom head ( a ) and healthy human volunteers ( b ). The electric stimulator was located outside the shielded MEG room and delivered 1 mA. The distance between the electric stimulation electrodes and the MEG sensor array (turquoise tubes) was 2–6 cm. Full size image Other important prerequisites to test the reliability of signal source reconstruction of brain oscillations during application of transcranial electric currents include the availability of ultra-stable electric current sources (current variance during stimulation <0.02% to allow well-controlled application of electric currents) and the use of recently developed radiotranslucent, non-ferrous, rubber-based stimulation electrodes that let neuromagnetic brain oscillations pass so that activity directly underneath the stimulation electrodes can be recorded. By utilizing these technical advances and combining them with synthetic aperture magnetometry (SAM) [30] , a mathematical approach offering intrinsic spatially-selective noise reduction and source localization, we developed a novel strategy that allows Transcranial Electric Stimulation during Assessment of Neuromagnetic Activity (TESANA). The reliability and robustness of this novel strategy was tested using an electrolyte-filled sphere (phantom head) with an oscillating dipole source inside. Stimulator-dependent electromagnetic noise levels were quantified. We then tested whether SAM is a robust tool to localize and reconstruct activity of an oscillating signal source in the presence of significant electromagnetic noise (>30 dB relative to sensor noise) generated by electrodes placed in the immediate proximity (2–6 cm) of the MEG sensor array, the usual distance for MEG recordings in human adults [31] . This approach was then tested in five healthy human volunteers by assessing task-related changes in brain oscillatory activity in the rolandic alpha (also called sensori-motor rhythm, SMR, 8–13 Hz) and beta (13–30 Hz) frequency bands recorded from motor cortical areas undergoing 1 mA anodal tDCS during a self-paced button-press task. Power spectra of brain oscillations during task-free intervals were computed in the absence of and during electric current stimulation to test for the generalizability of this novel strategy to other MEG signals. Additionally, generalization to other head locations was tested by embedding a set of simulated dipoles into the measured interference data at different head locations and quantifying reliability of their reconstruction. We found that characterization of changes in brain oscillatory activity and motor behavior during transcranial electric brain stimulation is now possible using this novel approach. Generalizability to other MEG signals (for example, task-free activity) and other head locations was successfully proven. Respecting the theoretical and practical limitations of the MEG system, our data suggest that this novel strategy can also be used with other stimulation protocols such as oscillating current stimulation or transcranial alternating current stimulation (tACS), and thus will allow development of a broad spectrum of applications in cognitive neuroscience and neuromodulation of brain function. Quantification of noise induced by tDCS Evaluation of noise characteristics of two different tDCS devices using the phantom head ( Fig. 1a ) indicated that both stimulators generated significant electromagnetic noise resulting in signal power changes up to 4 dB (relative to sensor noise) on average across the MEG sensor array (device A: 11.48 dB; device B: 4.01 dB). Noise was highest at lower frequencies and decreased by 6.70 dB per octave exhibiting the characteristic features of brown noise [32] . Noise levels were highest around the stimulating tDCS electrodes (device A: 30.6 dB, device B: 10.2 dB relative to sensor noise), but still detectable in areas remote from the stimulation electrode (>8 cm) ( Fig. 2 ). 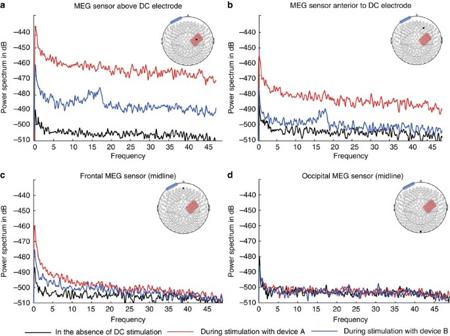Figure 2: Topographic illustration of signal power during different experimental conditions. Signal power is shown in absence of electric stimulation (black), during stimulation with device A (red) and device B (blue) using a phantom head. Noise levels as measured in a magnetoencephalography (MEG) sensor with the highest level of noise above the extracephalic stimulation electrode (a), anterior of the electrode (b), in the most frontal (c) and occipital (d) MEG sensor. While noise is strongest above the electrode during stimulation with device A (NeuroConn DC Stimulator Plus); device B (prototype of NeuroConn DC Stimulator nG) generates much less noise (a), decreasing with distance from the electrode (b,c). We used different stimulation devices to investigate whether robustness of TESANA depends on the magnitude of stimulator noise. Figure 2: Topographic illustration of signal power during different experimental conditions. Signal power is shown in absence of electric stimulation (black), during stimulation with device A (red) and device B (blue) using a phantom head. Noise levels as measured in a magnetoencephalography (MEG) sensor with the highest level of noise above the extracephalic stimulation electrode ( a ), anterior of the electrode ( b ), in the most frontal ( c ) and occipital ( d ) MEG sensor. While noise is strongest above the electrode during stimulation with device A (NeuroConn DC Stimulator Plus); device B (prototype of NeuroConn DC Stimulator nG) generates much less noise ( a ), decreasing with distance from the electrode ( b , c ). We used different stimulation devices to investigate whether robustness of TESANA depends on the magnitude of stimulator noise. Full size image Identification of the artificial dipole source is precise Activating the oscillating signal source inside the phantom head and employing SAM for source localization and reconstruction resulted in accurate characterization of the pre-determined source activity (mean deviation in mm: 4.17±2.88) (see Table 1 ). Accuracy of localization was stable and did not change with the onset of tDCS stimulation (one-way ANOVA, F (2,6)=0.02, P =0.98) ( Fig. 3a–c ). Table 1 Localization of the generated oscillating dipole signal. 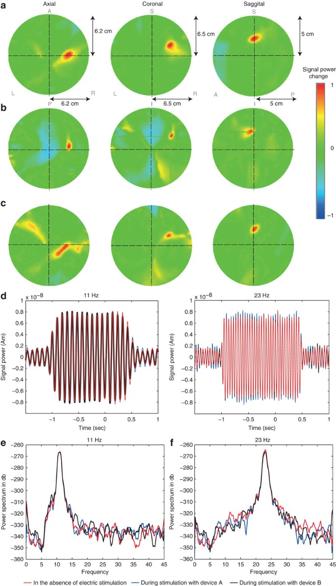Figure 3: Signal localization and reconstruction during and in absence of electric stimulation. Synthetic aperture magnetometry (SAM)-based localization of the generated oscillating dipole signal (5 Hz, 8 nAm) in absence (a) and during electric stimulation with device A (b) and device B (c) within the electrolyte-filled phantom head. Localization of the signal source characterized by the largest signal power changes (maximum in red) was consistent across conditions (a–c). (d) SAM-based reconstruction of the generated dipole signal oscillating at 11 Hz (left) and 23 Hz (right). Field strength of the dipole signal was changed from 3–10 nAm to resemble task-related changes of neuromagnetic oscillatory brain activity typically found in the human brain. Similarity between the generated and reconstructed signal source reflects the fidelity of TESANA. Frequency spectra (e) of recorded activity while the generated dipole signal was oscillating at 11 Hz (left) and 23 Hz (right) indicate a clear and undistorted power peak at the tested frequencies, and no stimulation specific distortions in other frequencies. Full size table Figure 3: Signal localization and reconstruction during and in absence of electric stimulation. Synthetic aperture magnetometry (SAM)-based localization of the generated oscillating dipole signal (5 Hz, 8 nAm) in absence ( a ) and during electric stimulation with device A ( b ) and device B ( c ) within the electrolyte-filled phantom head. Localization of the signal source characterized by the largest signal power changes (maximum in red) was consistent across conditions ( a – c ). ( d ) SAM-based reconstruction of the generated dipole signal oscillating at 11 Hz (left) and 23 Hz (right). Field strength of the dipole signal was changed from 3–10 nAm to resemble task-related changes of neuromagnetic oscillatory brain activity typically found in the human brain. Similarity between the generated and reconstructed signal source reflects the fidelity of TESANA. Frequency spectra ( e ) of recorded activity while the generated dipole signal was oscillating at 11 Hz (left) and 23 Hz (right) indicate a clear and undistorted power peak at the tested frequencies, and no stimulation specific distortions in other frequencies. Full size image TESANA results in undistorted reconstruction of oscillations The reconstructed signal at the identified location exhibited high coherence during electrical stimulation when compared with recordings in the absence of stimulation (device A: rolandic alpha and beta: 0.99±0.002; device B: alpha: 0.99±0.000; beta: 0.997±0.001) (see Table 2 and Figure 3d ). For validation of generalizability of the results at other head locations, localization and reconstruction of 11 simulated dipoles embedded into the interference data recorded in the presence of stimulation resulted in high coherence between conditions in all simulated dipoles (mean coherence: 0.9967+/−0.004, Supplementary Fig. S1 , Supplementary Table S1 ). Table 2 Coherence of signal reconstruction. Full size table Motor task-related changes of brain oscillations during tDCS Topographic field analyses of task-related changes in neuromagnetic activity during self-paced finger tapping motions of the left index finger in ‘sensor space’ indicated a central dipole source with the highest field strength around the time of the button press ( Fig. 4a ). This finding was consistent with numerous previous studies [33] . During active electrical brain stimulation, the dipole source could not be identified anymore ( Fig. 4b ). Stimulation-dependent artifacts were most pronounced in left and right anterior and central MEG sensors ( Fig. 4b ). 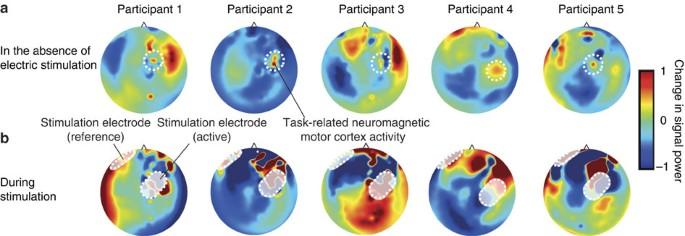Figure 4: Topographic maps of motor task-related signal power changes. Absolute signal power changes (0.5–30 Hz) during self-paced left index finger button presses across participants in the absence of stimulation (a) and during electric stimulation (b). Note the stimulation artefacts (dark red) superimposing task-related neuromagnetic motor cortex activity in the centro-parietal sensor space (white dotted circle). Figure 4: Topographic maps of motor task-related signal power changes. Absolute signal power changes (0.5–30 Hz) during self-paced left index finger button presses across participants in the absence of stimulation ( a ) and during electric stimulation ( b ). Note the stimulation artefacts (dark red) superimposing task-related neuromagnetic motor cortex activity in the centro-parietal sensor space (white dotted circle). Full size image SAM-based analyses computing neuromagnetic dipole activity in an assumptive ‘source space’ and co-registering such space with actual anatomical data of each individual localized the voxel with the most significant task-related signal source change in the primary motor cortex (M1, Brodman area 4) ( Fig. 5a ). Localization was not influenced by active tDCS (average deviation: 4.56±2.89 mm) ( Fig. 5b ), and results matched with findings in other neuroimaging studies [34] , [35] . Task-related signal source changes (for example, rolandic alpha desynchronization before or beta synchronization after button press) in the absence of and during DC stimulation ( Fig. 6a–e ) were consistent with previous results in studies that extensively investigated motor-related changes of brain oscillatory activity [36] , [37] . Further frequency-specific analyses of changes in alpha and beta power values indicated no significant differences between runs recorded in the absence of and during electrical brain stimulation (alpha pre-button-press: T(4)=−0.338, P =0.563; alpha post-button press: T(4)=−0.696, P =0.525; beta pre-button-press: T(4)=−0.338, P =0.753; beta post-button press: T(4)=0.332, P =0.757). Comparison of power spectra of task-free activity in M1 during and in absence of stimulation showed no significant distortions ( Fig. 6 , right column). 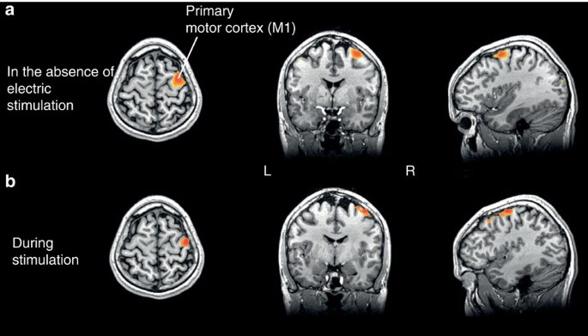Figure 5: Localization of motor task-related signal changes. The voxels with the most significant task-related signal source change in the range of 0.5–30 Hz during self-paced button pressing (here of participant 1 for illustration) were reliably localized in the primary motor cortex (M1, Brodman area 4) irrespective of the absence (a) or presence of electric stimulation (b). In (b) electric stimulation was applied by a radiotranslucent, non-ferrous electrode placed over M1. Figure 5: Localization of motor task-related signal changes. The voxels with the most significant task-related signal source change in the range of 0.5–30 Hz during self-paced button pressing (here of participant 1 for illustration) were reliably localized in the primary motor cortex (M1, Brodman area 4) irrespective of the absence ( a ) or presence of electric stimulation ( b ). In ( b ) electric stimulation was applied by a radiotranslucent, non-ferrous electrode placed over M1. 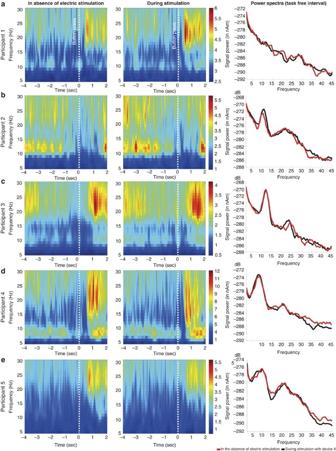Figure 6: Cross-frequency spectrum of brain oscillations during a motor task. Cross-frequency spectrum of self-paced left index finger button press-related signal source changes in the primary motor cortex (M1) in absence (left) and during (middle) electric stimulation across all participants (a–e). Note the typical motor task-related changes of signal power in alpha (8–13 Hz) (alpha desynchronization shortly before and after button press; most prominent in participants 2 and 4) and beta (13–30 Hz) (beta synchronization approximately one second after the button press) as described by Pfurtscheller and Aranibar37and others. Frequency spectra of MEG activity during task-free intervals (right) exhibit the typical physiologic alpha and beta peaks, and indicate no stimulation specific distortions in other frequencies. Full size image Figure 6: Cross-frequency spectrum of brain oscillations during a motor task. Cross-frequency spectrum of self-paced left index finger button press-related signal source changes in the primary motor cortex (M1) in absence (left) and during (middle) electric stimulation across all participants ( a – e ). Note the typical motor task-related changes of signal power in alpha (8–13 Hz) (alpha desynchronization shortly before and after button press; most prominent in participants 2 and 4) and beta (13–30 Hz) (beta synchronization approximately one second after the button press) as described by Pfurtscheller and Aranibar [37] and others. Frequency spectra of MEG activity during task-free intervals (right) exhibit the typical physiologic alpha and beta peaks, and indicate no stimulation specific distortions in other frequencies. Full size image This is the first study demonstrating the feasibility of identifying changes in oscillatory brain activity during non-invasive electrical brain stimulation. The effects of tDCS are well documented in the behavioral and cognitive domain [14] , [15] , [16] , [22] , [38] . However, the online effects of electrical brain stimulation on a millisecond-by-millisecond scale of human brain physiology are not known [39] . Here, we introduced a strategy that allows for millisecond-by-millisecond in vivo investigation of changes in pattern formation of neural cell assemblies’ activity and evaluation of changing functional connectivity during exctracephalic electric current stimulation. While application of tDCS is associated with significant electromagnetic noise, which peaks in close proximity to the electrodes ( Figs 2 , 4 ), we demonstrated elimination of such noise and accurate characterization of neuromagnetic oscillatory activity, despite proximity to the electrodes. Neuromagnetic activity passing the radiotranslucent, non-ferrous electrodes resulted in reliable localization and reconstruction of signal sources ( Fig. 5 ). Self-paced button press-related changes of neuromagnetic activity in alpha and beta frequencies during electric stimulation were not different from measurements recorded in the absence of externally applied electric currents ( Fig. 6 ). The robustness of TESANA was independent of the electrical stimulator’s noise characteristics as two devices exhibiting different characteristics were tested. Acquisition of neuromagnetic activity during tDCS using a whole-head MEG proved practical and safe. Recorded neuromagnetic activity was unaffected by radiotranslucent electrodes and allowed further processing of the cortical dipole sources directly underneath the stimulation site on the skull. This study, which was designed to evaluate a novel strategy allowing simultaneous electric brain stimulation during whole-head MEG recordings, was not powered to relate this activity with previously demonstrated changes of brain excitability [13] or motor behavior [15] , an issue of interest for future investigations. Besides SAM-based beam-forming, other techniques such as signal space separation [40] or minimum norm [41] shown to be advantageous in the reconstruction of correlated sources [42] or minimizing leakage [43] , might complement SAM beam forming. However, while signal space separation is a noise-reduction algorithm without providing source localization, minimum norm does not constitute an adaptive solution and must be used in conjunction with additional methods for interference reduction such as ICA that increases the risk for mis-localization in the presence of interference. Apart from tDCS, other stimulation protocols also showed to have specific effects on brain function and behavior, for example, transcranial oscillating current stimulation [44] , tACS [45] or random noise stimulation [46] . Our data and consideration of theoretical boundaries suggest that this new strategy can be generalized to other stimulation protocols as long as the electromagnetic interference from the stimulator does not exceed the dynamic recording range and maximum slew rate of the MEG system. Strong magnetic fields close to the SQUIDS can cause magnetic flux trapping [47] , an issue that requires caution, as degradation of the SQUID sensors can result. The MEG that was used for the study was a CTF 275-sensor whole-head MEG system with a dynamic recording range of 192 dB. This system employs a digital flux-locked loop that allows for slew rates of up to 36.000 Φ 0 s −1 (Φ 0 equals one flux quantum). Based on a sensor gain of 3.25 × 10 −16 T per bit, the theoretical bounds for this device are therefore 6.13 μT s −1 . Given a current intensity of 1 mA generating a magnetic field with a peak signal value of ~5 nT, a maximum frequency of 195 Hz would be possible (see Supplementary Methods ), allowing frequency-tuned tACS [48] at any previously investigated frequency. To our knowledge, no stimulation protocol previously tested in human non-invasive electrical brain stimulation (except high-frequency RNS [46] with frequency peaks of up to 640 Hz) exceeds these theoretical boundaries. This novel technique for the in vivo assessment of brain oscillations during transcranial electric brain stimulation promises to make important contributions towards a better understanding of the effects of non-invasive electric current stimulation on brain function and behavior. An important advantage of this novel strategy is that it mainly combines existing materials, devices and mathematical models for a new use, allowing fast implementation in other laboratories. Findings resulting from this novel strategy may allow for enhanced and more individualized brain-stimulation-based treatment strategies for patient populations suffering from a wide variety of neurological or psychiatric disorders, including stroke, depression, chronic pain or schizophrenia [49] . Finally, recent studies have demonstrated that beam forming can be used in online brain–computer interfaces (BCI) translating neuromagnetic signals into control signals of external devices [50] . Such paradigms allow for learned control of brain activity of specific cortical and subcortical areas [51] . The combination of BCI systems and TESANA, as introduced here, might be a new way to modulate BCI control through brain-state-dependent electrical stimulation non-invasively and to establish a bidirectional BCI or brain–machine–brain interface [52] previously described in an invasive setup. Artificial sensory feedback was applied by intracortical microstimulation enabling a monkey to ‘feel’ when an actuator (in this case, a virtual reality arm) touched a virtual object [52] . Our results suggest that such a paradigm might be also feasible non-invasively. Future studies investigating the application of brain-state dependent transcranial electric currents during MEG-based BCI control may result in new strategies in the restoration of brain function (neurorestoration). Magnetoencephalography Magnetoencephalography (MEG) is optimally designed to identify the timing and direction of currents and is thus an ideal tool for reconstructing and localizing oscillating signal sources with superior temporal and spatial resolution [53] , [54] , as shown by the reliable mapping of signal sources in the sensory, motor, visual and auditory cortices [55] . Magnetic signals were recorded at 600 Hz with a bandwidth of 0–150 Hz using an MEG instrument with a whole-head array comprising 275 radial first order gradiometer/SQUID channels (CTF MEG by MISL, Coquitlam, Canada) housed in a magnetically shielded room (Vacuumschmelze, Germany). Synthetic third gradient balancing was used to remove online background noise. Phantom dipole model A spherical phantom head with a diameter of 13 cm containing two electrodes and filled with a saline electrolyte solution was used to generate an oscillating dipole at a fixed location relative to the center of the sphere (coordinates [−40 mm, 0 mm, 25 mm] according to RAI) ( Fig. 1a ). The dipole-generating electrodes had an inter-electrode distance of 4 mm. The dipole signal was set to oscillate at different frequencies (11 and 23 Hz) and reconstruction was tested during variable activity (at 3–10 nAm source strength) to resemble task-related changes of brain oscillatory activity. Participants Five healthy human volunteers (three male, two female, 28±5.8 years old; all right-handed) without a history of neurological or psychiatric disorders participated in this study. The study was approved by the ethics committee of the Medical Faculty at the University of Tübingen. All studies were carried out at the University of Tübingen. Before the first MEG measurement, the location of M1 was assessed by single-pulse transcranial magnetic stimulation according to Rossini et al. [56] and marked with a water-resistant skin marker. Three fiducial localization coils were placed at the nasion and pre-auricular points (right and left) to determine the head position in real time during MEG recordings. Before each measurement, coil positions were photographed for offline co-registration of the recorded MEG data with structural T1 MR images. MRI images A cranial MRI exam in a 3-T whole-body scanner with a 12-channel head coil (Magnetom Trio, Siemens, Erlangen, Germany) was carried out, while the participants were placed supine in the scanner. Vitamin E capsules served as radiological markers for the nasion and pre-auricular points corresponding to locations used for MEG head localization. T1-weighted structural scan of the whole brain were obtained using the sequence MPRAGE (matrix size=256 × 256, 160 partitions, 1 mm [3] isotropic voxels, TA=5:17 m, TR=2300, ms, TE=3.93 ms, flip angle=8°, FOVRO=256, FOVPE=224, PAT=2, PAT mode=GRAPPA) and served as the anatomical reference. Electric brain stimulation Direct current was applied to the phantom head using a commercial and a prototype stimulator (NeuroConn GmbH, Ilmenau, Germany). The radiotranslucent stimulator electrodes were placed in a bipolar montage over C4 (stimulating electrode) and below FP1 (reference electrode) according to the International 10–20 system ( Fig. 1a ), and had a size of 6 × 4 cm. The battery-driven stimulator device was located outside the magnetically shielded room and delivered electric currents via a twisted pair of wires with an intensity of 1 mA. A conductive paste (Ten20, D.O. Weaver, Aurora, CO, USA) was applied to the surface of the phantom, allowing a constant current flow between the electrodes at impedance values of 8–12 kΩ matching the values of a real head. This allowed for quantification of stimulator-dependent electromagnetic noise levels as well as changes in the reconstructed signal source compared with the predefined location and oscillating activity of the dipole. As due to the low conductivity of the skull (5.52 × 10 −3 S/m) [57] only a fraction of the applied currents enter the head, this phantom model was considered most appropriate compared with other models, for example, the use of an agar sphere. Two different stimulator devices with different noise characteristics were tested separately (device A: DC Stimulator plus and device B: a new stimulator prototype/DC Stimulator nG, both NeuroConn GmbH). Electromagnetic noise recorded by the MEG sensor array was evaluated by computing the power spectrum for all MEG channels in the absence of any oscillating dipoles. The same stimulator (device A) and stimulation electrodes were used for the experiments with healthy human volunteers. Electrodes were placed in a bi-cephalic montage (anode placed over the right M1, reference electrode placed to the supraorbital area; Fig. 1b ). Recordings in absence of stimulation were conducted without the stimulating electrodes in place, to allow proper validation of the control condition. For tDCS, electric currents were gradually ramped up from 0.0–1.0 mA over 15 s and kept constant until all 60 self-paced button presses were completed. Impedance levels of the tDCS electrodes were kept below 12 kΩ. Self-paced button press task during MEG recordings All participants were seated upright in the shielded MEG room with their hands placed on a cushion on their laps and their head centrally positioned within the MEG sensor array. A closed-circuit video system was used to constantly monitor the experiment, while instructions were given during rest periods via an intercom system. The participants were instructed to voluntarily press a button placed under the left index finger with a time interval of at least 8–12 s between each press. After collecting MEG data during three runs with 60 button presses in the absence of electric brain stimulation, recordings continued, while anodal tDCS was delivered by device A (3 runs, 60 button presses). Offline analysis Electromagnetic noises generated by device A and device B were evaluated for every MEG sensor and averaged across the whole MEG sensor array. Changes in sensor signal power were topographically mapped. A Fourier transformation of the MEG signals recorded from four different locations in the MEG sensor array (above the stimulating tDCS electrode, anterior to the stimulating electrode, one frontal and one occipital midline MEG sensor) was performed for data acquired in the absence of tDCS and during tDCS with devices A and B. Fourier transformations were also performed for MEG data recorded during simulation of the 11 and 23 Hz dipoles and during task-free intervals (−4 to −2 s before button presses) in all tested healthy participants. Statistical analysis All data are presented as mean ±s.d. and were analyzed using a two-tailed Student’s t -test or one-way ANOVA. Statistical significance was set at P <0.05 and is indicated on figures with an asterix (*). The specific text, P -value and F-statistics (ANOVA) for each comparison are described in the Results section. Source reconstruction using SAM Source reconstruction was performed using SAM, a scalar linearly constrained minimum variance beam former acting as a spatial filter for estimating cortical source activity on a voxel–by-voxel basis (see Supplementary Methods ). Source power was calculated at 1-mm intervals on a regular three-dimensional grid throughout the phantom head. A dual-state SAM analysis included a nonparametric U -test to identify the location of the voxel with the most significant amplitude change. A second order Butterworth band-pass filter was applied with cutoff frequencies of 8 and 15 Hz for the simulated 11 Hz signal source and 15 and 30 Hz for the simulated 23 Hz signal source, respectively. A one-way ANOVA was used to test for differences in accuracy of source localization (as measured by deviation from the given coordinates of the simulated dipole) and coherence of source reconstruction. Coherence, a measure of similarity between two given signals [58] , was quantified using the following equation. where P xy is the cross power spectral density and P xx and P yy , the power spectral density of each signal, x and y , respectively. For all statistical tests, the significance level was set to P <05. MEG data recorded from healthy human volunteers was band-pass-filtered with cutoff frequencies between 0.5 and 30 Hz and segmented into epochs of 2 s based on button-press-related trigger markers. Task-related changes in alpha and beta frequencies were quantified in sensor space for time windows of 1 s before and 1 s after the button presses. Signal changes were averaged across all epochs in the absence of and during tDCS, and topographically displayed. For signal source reconstruction and localization in source space, MEG data was co-registered using the radiological markers in the participant’s T1-weighted MR images and the MEG fiducial coil coordinates. A time-frequency analysis was performed using a multitaper spectral method [59] implemented in Fieldtrip [60] . Signal power in alpha (8–13 Hz) and beta (13–30 Hz) were computed for 1-s time windows 0.5 s before button-press and 1 s after button press, and compared between runs recorded in the absence of and during DC stimulation using a paired-samples t -test. How to cite this article: Soekadar, S R. et al. In vivo assessment of human brain oscillations during application of transcranial electric currents. Nat. Commun. 4:2032 doi: 10.1038/ncomms3032 (2013).